Generation of 1020W cm−2hard X-ray laser pulses with two-stage reflective focusing system Intense X-ray fields produced with hard X-ray free-electron laser (XFEL) have made possible the study of nonlinear X-ray phenomena. However, the observable phenomena are still limited by the power density. Here, we present a two-stage focusing system consisting of ultra-precise mirrors, which can generate an extremely intense X-ray field. The XFEL beam, enlarged with upstream optics, is focused with downstream optics that have high numerical aperture. A grating interferometer is used to monitor the wavefront to achieve optimum focusing. Finally, we generate an extremely small spot of 30 × 55 nm with an extraordinary power density of over 1 × 10 20 W cm −2 using 9.9 keV XFEL light. The achieved power density provides novel opportunities to elucidate unexplored nonlinear phenomena in the X-ray region, which will advance development on quantum X-ray optics, astronomical physics and high-energy density science. X-ray free-electron laser (XFEL) light sources have been used to generate intense X-ray pulses. The FLASH facility in Germany [1] , the SPring-8 Compact SASE Source test accelerator in Japan [2] and FERMI in Italy [3] have successfully generated soft X-ray lasers. The Linac Coherent Light Source in the US achieved the first ever lasing in the hard X-ray region [4] . The SPring-8 Angstrom Compact Free-Electron Laser (SACLA) produced the shortest ever wavelength laser, achieving operation in the 0.6 angstrom wavelength range [5] . An important characteristic of X-rays is their capability to be focused down to a nanometer-sized spot due to their short wavelength. The diffraction-limit theory based on the fundamental nature of light states that the wavelength governs the minimum resolution in imaging and focusing techniques. This decade, X-ray focusing devices have significantly progressed and some devices have reached their diffraction limited performance [6] , [7] producing focal beam sizes of 10 nm [8] , [9] . Such focusing optics are able to enhance the characteristics of XFEL light by increasing power density [10] , [11] , [12] , which is highly desirable for investigating interactions between X-rays and matter [13] , [14] . In order to realize a smaller spot size, a smaller focal distance and larger aperture are required, following the diffraction-limit theory [15] . However, a small focal distance imposes a serious problem on most experiments using intense XFEL, because debris from the target, produced by the irradiation of the XFEL pulses, could severely degrade the optical performance. A larger incident beam size is necessary to reduce the focus size; however, this is difficult to achieve due to the divergence of the XFEL beam, which is in the order of microradians. To overcome this difficulty, we develop a two-stage focusing system comprising a pair of focusing mirrors in the Kirkpatrick Baez geometry [16] at SACLA. The focal beam size is estimated by the wave optical simulation, optimized with grating interferometry and directly measured by the knife-edge scan method. Finally, we successfully generate 10 20 W cm −2 hard X-ray laser pulses with a beam spot of 30 nm × 55 nm using 9.9 keV XFEL light. 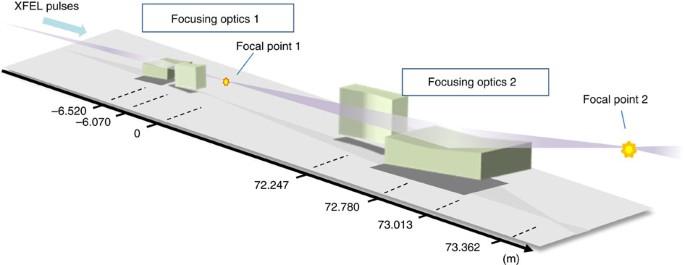Figure 1: Two-stage reflective focusing system. The XFEL pulse is optimally magnified once by the upstream focusing system and efficiently focused by the downstream focusing system with a high numerical aperture using two Kirkpatrick Baez geometries. This system is installed in the SACLA. Optical system Figure 1 shows two-stage reflective focusing system installed in BL3 of SACLA. We use a new scheme that utilizes a pre-focusing system that forms a small source and effectively expands the beam size at the final focus [17] (see Methods).Utilization of total reflection optics enabled us to cover a wide range of wavelengths. Detailed optical parametres are listed at Table 1 . At the expense of increased divergence of the focused beam, we designed the optical system with the smallest possible beam size to increase the power density. Four mirrors were precisely fabricated by deterministic figure correction processes consisting of elastic emission machining (EEM) and interferometric metrology (see Methods) [18] , [19] , [20] . The figure accuracy and the surface roughness achieved were 2 nm (peak-to-valley) and 0.2 nm (root mean squared), respectively [7] , [10] . The first pair of focusing mirrors was placed 120 m downstream from the end of the undulator to focus the XFEL pulses to a spot of ~3.6 μm (vertical) × 3.2 μm (horizontal) with nearly 100% efficiency [10] . The diverged XFEL beam propagates to the second pair of focusing mirrors, which was located ~72 m downstream from the upstream device. For the final focusing optics, a large aperture size of 2.3 mm × 2.7 mm was realized using 465-mm and 500-mm-long substrates coated with platinum that have large critical angles. The ideal beam size defined as the full width at half maximum (FWHM) of the intensity profile was ~30 nm and 55 nm at 10 keV in the vertical and horizontal directions, respectively, with a long working distance of 350 mm. These sizes were calculated by considering both the XFEL source size and the optical geometry of the focusing system [10] . Figure 1: Two-stage reflective focusing system. The XFEL pulse is optimally magnified once by the upstream focusing system and efficiently focused by the downstream focusing system with a high numerical aperture using two Kirkpatrick Baez geometries. This system is installed in the SACLA. Full size image Table 1 Optical parameters of designed focusing mirrors. Full size table Although the four-mirror system significantly improves performance theoretically, mirror alignments to achieve optimum focusing are necessary. Furthermore, the wavefront information, in addition to the focusing profile, could play an important role in applications [21] . Therefore, we have developed a grating interferometer utilizing the Talbot effect, which enables us to obtain wavefront profiles [22] , [23] . The phase grating near the focus produces striped interference fringe patterns at a specific distance downstream from the grating. The irregular patterns imply that the wavefront of the XFEL pulses is distorted. Inverse calculations using the Fourier transform method reproduce the wavefront profiles (see Methods). Since the grating is placed outside the focus, the wavefront profiles can be monitored in situ . XFEL focusing experiment An XFEL-focusing experiment was performed at 9.9 keV with a bandwidth of 50 eV (FWHM) that was measured by scanning a double crystal monochromator with Si(111) [24] . 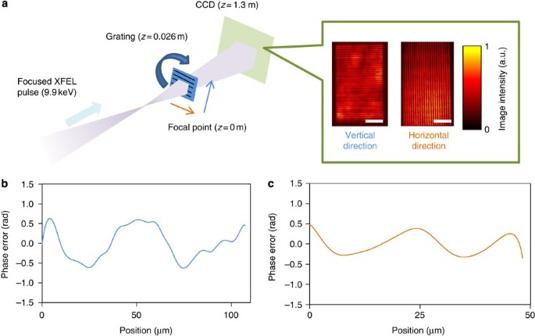Figure 2: Wavefront measurement by grating interferometry. The wavefront profiles measured in the vertical and horizontal directions are displayed separately. They are calculatedin situand can be used for mirror alignment. (a) Schematic drawing of the experimental layout. (b) Phase error profile of the focused beam on the grating plane in the vertical direction. (c) Phase error profile on the grating plane in the horizontal direction. Scale bars, 1 mm (in CCD images ofa). Figure 2a shows a schematic drawing of the single-grating interferometry setup. Parametres in detail are listed in Table 2 . The grating and a CCD camera were set 26 mm and 1.3 m downstream of the focal point, respectively. After the grating was inserted into the beam path, a striped interference pattern was observed with the CCD camera. Two gratings were prepared to evaluate the wavefront in the vertical and horizontal directions independently. Only single XFEL pulse was utilized for the detection of the interference images. Figure 2b,c show the estimated wavefront error profiles of the focused XFEL pulses in the vertical and horizontal directions, respectively. After precise alignment, the wavefront errors decreased and finally reached a sufficiently small value of 1 rad. Figure 2: Wavefront measurement by grating interferometry. The wavefront profiles measured in the vertical and horizontal directions are displayed separately. They are calculated in situ and can be used for mirror alignment. ( a ) Schematic drawing of the experimental layout. ( b ) Phase error profile of the focused beam on the grating plane in the vertical direction. ( c ) Phase error profile on the grating plane in the horizontal direction. Scale bars, 1 mm (in CCD images of a ). Full size image Table 2 Parameters of grating interferometer. 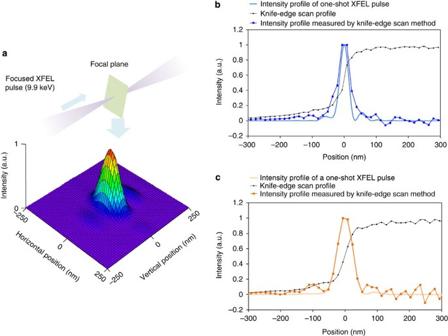Figure 3: Intensity profile of focused XFEL pulse. The intensity profiles on the focal plane are estimated when the wavefront of the focused beam is as shown inFig. 2. They are also measured by the knife-edge scan method. The estimated beam size is 30 nm (FWHM) in the vertical direction and 55 nm (FWHM) in the horizontal direction. (a) Estimated shape of intensity profiles on the focal plane. (b) Intensity profile in the vertical direction. (c) Intensity profile in the horizontal direction. Full size table Figure 3 shows the intensity profiles on the focal plane, which were evaluated considering the wavefront errors. The focused beam size was determined to be 30 nm × 55 nm, which was almost the same as that estimated under ideal conditions. The intensity profiles were also measured with a conventional knife-edge scan method. Twenty XFEL pulses were accumulated during the measurement of intensity for each stage position [10] . The beam size was 45 nm × 55 nm, which is larger than that evaluated by grating interferometry in the vertical direction. This discrepancy may result from the mechanical instability of the mirrors that is ~25 nm in amplitude in this direction. Figure 3: Intensity profile of focused XFEL pulse. The intensity profiles on the focal plane are estimated when the wavefront of the focused beam is as shown in Fig. 2 . They are also measured by the knife-edge scan method. The estimated beam size is 30 nm (FWHM) in the vertical direction and 55 nm (FWHM) in the horizontal direction. ( a ) Estimated shape of intensity profiles on the focal plane. ( b ) Intensity profile in the vertical direction. ( c ) Intensity profile in the horizontal direction. 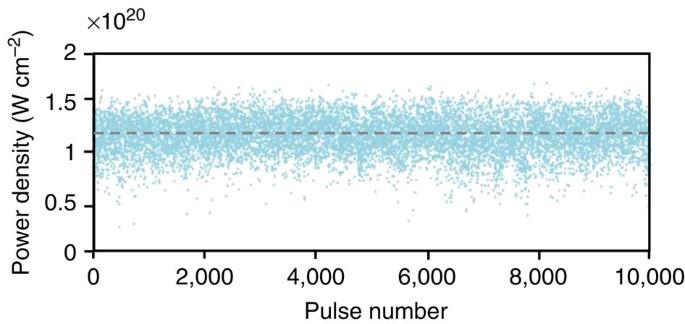Figure 4: Estimated power density of each XFEL pulse on focal plane. The X-ray energy is 9.9 keV. The pulse duration is 7 fs. The average energy of the XFEL pulses entering the downstream focusing optics is 42 μJ. The reflectivity value of the vertical and horizontal mirrors is ~88%. The percentage of reflected X-rays within the FWHM is 34%. The FWHM of the beam profile is 30 × 55 nm. Full size image Power density Figure 4 shows the power densities estimated at the focal point, using the beam shape shown in Fig. 3 . The pulse duration was assumed to be 7 fs [24] . The power of each XFEL pulse can be precisely evaluated using the pulse energies measured with a backscattering beam monitor [25] , which gave an averaged pulse energy of 11 μJ per pulse at the focus in an experiment. These experimental results show that the average power density achieved was at least 1.2 × 10 20 W cm −2 at the focal plane (See Methods). Furthermore, we note that since the temporal intensity profile of XFEL pulses is a spike train [24] , the peak power density could be a few times higher than the average one. Figure 4: Estimated power density of each XFEL pulse on focal plane. The X-ray energy is 9.9 keV. The pulse duration is 7 fs. The average energy of the XFEL pulses entering the downstream focusing optics is 42 μJ. The reflectivity value of the vertical and horizontal mirrors is ~88%. The percentage of reflected X-rays within the FWHM is 34%. The FWHM of the beam profile is 30 × 55 nm. Full size image Recently, XFELs have stimulated progress in the field of nonlinear X-ray optics [13] , [14] , although the detectable nonlinear phenomena are still limited by the power density. One of the main reasons why the observation of multi-photon processes is disturbed is the ultra-short decay time of atoms after excitation with X-rays. For example, the relaxation time of the K-shell core hole that follows the photo absorption process is of sub-femtosecond order for 10-keV X-rays [14] . From simple evaluation, it is apparent that the intensity of 10 18 W cm −2 that has been realized with conventional schemes can excite only a certain percentage of atoms. By applying the intensity of 10 20 W cm −2 achieved in this work; however, we achieved conditions in which excited states dominate, realizing various nonlinear phenomena including the amplification of X-rays in simple solid targets, coherent scattering processes and ultrafast X-ray gating. Finally, it should be emphasized again that the focused spot size of the two-stage focusing system is highly tunable over a wide range of sizes, from nanometer to micrometer scales, while maintaining high efficiency and compact configuration. This unique character is highly useful for developing applications using brilliant synchrotron sources, such as coherent diffraction imaging, ptychography and photon correlation spectroscopy. Mirror fabrication process The substrate material of the four mirrors is quartz glass. First, the substrates were roughly machined by conventional grinding and polishing methods. Then, elliptically curved surface was completed using a computer controlled machining system consisting of EEM [18] and interferometric surface profilers [19] , [20] . EEM has a controllability of 0.1 nm in removing the surface material. The surface profilers were specially developed for measuring long X-ray focusing mirrors. The surface figure accuracy achieved was 2 nm in peak-to-valley over entire area of the long X-ray focusing mirrors [7] , [10] . Two of the mirrors of downstream focusing system are coated with platinum by magnetron sputtering. Geometrical optics of two-stage focusing In geometrical optics, following the thin-optics approximation, the focused beam size ( D 2 ) of lens 1 is given by where f 3 and f 4 are the focal distance and the distance between lens 1 and the source, respectively. D 3 is the source size. When the two-stage focusing system consists of lenses 1 and 2, the final focused beam size D 1 is where f 1 and f 2 are the focal distance of lens 2 and the distance between lens 2 and the focal point of lens 1, respectively. The position of the focusing optics that corresponds to f 4 is fixed following the beam path geometry. The focal distance f 1 should be relatively long. However, the focal spot size is reduced by increasing the ratio of f 2 to f 3 (ref. 17 ). Grating interferometry In this experiment, single-shot metrology was employed for determining the wavefront error of XFEL pulses. Two gratings with a micrometer pattern are set near the focal point. These gratings act as a phase shifter. The wavefront profile of the X-rays after passing through the gratings is striped. At a specific distance, distinct intensity patterns are formed, which provide information on the wavefront error of the diverging X-ray beam [22] . Wavefront profiles can be calculated by the Fourier transform method using the intensity distribution of one-shot XFEL pulses. They are measured in the vertical and horizontal directions separately. The parameters considered are listed in Table 2 . In a previous study [23] , the accuracy of a measured wavefront profile was confirmed to be in the order of 0.1 λ. Estimation of power density The average energy of the XFEL pulses entering the downstream focusing optics is 42 μJ in this estimation. The pulse duration was assumed to be 7 fs. Then, the reflectivity of the vertical and horizontal mirrors, which is the ratio of inserted to reflected photons, is ~88%, when the surface roughness is 0.2 nm (RMS). The focusing efficiency is defined as the percentage of X-rays gathering inside FWHM against the total X-rays reflected on the most downstream mirror. In the knife-edge scan method, the knife edge crosses through the focused beam with increasing blocking area in the focused beam. The focusing efficiency is directly determined by using the incident photon number [7] , [10] . The knife-edge scan profiles in Fig. 3 indicated that the focusing efficiency exceeded at least 34%. These experimental results show that the average power inside the FWHM is 11 μJ and the density achieved is 1.2 × 10 20 W cm −2 at the focal plane. How to cite this article : Mimura, H. et al. Generation of 10 20 W cm −2 hard X-ray laser pulses with two-stage reflective focusing system. Nat. Commun. 5:3539 doi: 10.1038/ncomms4539 (2014).